Direct observation of many-body charge density oscillations in a two-dimensional electron gas Quantum interference is a striking manifestation of one of the basic concepts of quantum mechanics: the particle-wave duality. A spectacular visualization of this effect is the standing wave pattern produced by elastic scattering of surface electrons around defects, which corresponds to a modulation of the electronic local density of states and can be imaged using a scanning tunnelling microscope. To date, quantum-interference measurements were mainly interpreted in terms of interfering electrons or holes of the underlying band-structure description. Here, by imaging energy-dependent standing-wave patterns at noble metal surfaces, we reveal, in addition to the conventional surface-state band, the existence of an ‘anomalous’ energy band with a well-defined dispersion. Its origin is explained by the presence of a satellite in the structure of the many-body spectral function, which is related to the acoustic surface plasmon. Visualizing the corresponding charge oscillations provides thus direct access to many-body interactions at the atomic scale. Interference is a general phenomenon that appears whenever we are dealing with the superposition of coherent waves. Because of the wave-particle duality, electrons can interfere as shown by Davisson and Germer [1] . The invention of the scanning tunnelling microscope [2] (STM) allowed the visualization of this effect in the real space by looking at the spectacular standing wave patterns produced by elastic scattering of electrons and holes at surface defects, such as vacancies, adsorbates, impurities or step edges [3] , [4] , [5] , [6] . These waves, known as Friedel oscillations [7] , correspond to modulations of the electronic local density of states [8] (LDOS) and can be energetically resolved by differential conductivity (d I /d U ) maps, usually measured at low temperature to reach a large coherence length and an improved energy resolution. This so-called quasi-particle interference (QPI) mapping was applied to several systems superconductors [9] being one of the most remarkable examples. Recently, it has been further expanded to study spin-split surface states on surface alloys [10] and topological insulators [11] , [12] . QPI has proven to be a powerful method to analyse electronic properties, such as energy dispersion relations [13] , lifetimes [14] , [15] , [16] , scattering phase shifts [1] , [7] , coherence lengths [9] and scattering channels [10] , [11] , [12] . One of the fundamental aspects of the QPI mapping is that in real space the amplitude of the LDOS oscillations reduces as the tip is moved away from the scattering centres. In part, this reduction is due to many-body inelastic decay [14] , [15] , [16] , since the injected quasiparticle, after a typical lifetime of several femtoseconds [17] (1 fs=10 −15 s), eventually relaxes into states closer to the Fermi level E F . In reciprocal space, this finite lifetime results in a broadening of the peaks related to the LDOS oscillation wavevectors in Fourier transformed (FT) QPI maps [18] . Although energy-relaxation mechanisms have been theoretically intensively investigated [19] , experimentally they are usually summarized within a single parameter: the aforementioned lifetime [17] , which corresponds to a non-zero imaginary part of the quasiparticle self-energy. To investigate many-body effects in more detail, recent experimental and theoretical efforts aimed at using QPI to probe both the real and imaginary part of the self-energy, an approach which allowed to visualize the presence of band-dispersion renormalization effects [20] , [21] , [22] . In particular, it was shown that the self-energy can be extracted by analysing both the dispersion and the width of the peaks in the FT QPI maps. However, the processes triggered by self-energy effects beyond the quasiparticle picture, that is, when apart from the Lorenz-type quasiparticle peak the many-body spectral function has other low-intensity features, and their influence on the local electronic properties always escaped experimental detection. Furthermore, the QPI maps do not only correspond to the LDOS oscillations but also contain a background contribution, which is thought to be proportional to the tunnelling current (see refs 23 , 24 ). The question of how the inelastic decay process can affect this background term of resulting QPI maps has not been addressed so far. Here, using STM measurements, we visualize how the Fermi sea locally rearranges to minimize the perturbation created by low-energy excitations. By analysing the QPI patterns produced around point defects at Cu, Ag and Au (111) surfaces, we provide evidence that the two-dimensional (2D) electron gas exhibits an additional contribution to the LDOS oscillations, which leads to extra modulations in the QPI and are related to the acoustic surface plasmon [25] , [26] (ASP). For this contribution, systematic energy-dependent measurements reveal a well-defined energy-wavevector dispersion relation that is determined by the detailed structure of the many-body spectral function of a quasiparticle in the surface-state band. We also show that the so-called secondary electrons and holes incoherently produced during the inelastic decay process of an injected quasiparticle can contribute to the formation of QPI patterns as well. These secondary quasiparticles generate self-interfering patterns, which are cumulated to form the background contribution. We believe that our findings further expand the capabilities of QPI mapping as an experimental technique to study many-body effects in condensed matter physics. Experimental observations We have studied the (111) surfaces of the noble metals Cu, Ag and Au, which are known as model systems for a 2D electron gas (2DEG) due to the existence of a partially occupied s – p -derived surface state in the bulk L -gap [27] . Although usually described within a single-particle approach, these systems are known to exhibit relevant many-body effects, being plasmons the most prominent example [28] . At the same time, they are simple enough for a precise theoretical description allowing a direct comparison with experiments. 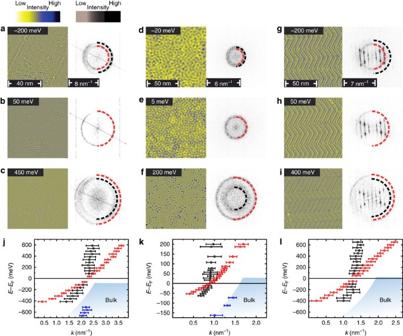Figure 1: Spectroscopic mapping of charge waves. (a–i) dI/dUmaps with respective FT images obtained at different energies on Cu, Ag and Au. Two distinct rings in FT images merging into a single one at energies close toEFare visible on all three surfaces. Low row shows energy-wavevector dispersion relations of two rings for (j) Cu, (k) Ag and (l) Au. Data have been obtained by analysing the FT QPI pattern at different energies. Red points correspond to the surface-state dispersion. Black points correspond to the additional oscillations with wavevector denoted askEH. Below the onset of the surface states, wavevectors corresponding to bulk states can be detected for Cu and Ag. The error bars have been calculated according to the procedure described in the Methods section. Figure 1 presents d I /d U maps obtained for Cu, Ag and Au at different energies. The corresponding Fourier transformations translate the real space information into the reciprocal space, thereby providing a convenient way to analyse the wavevector of the LDOS oscillations as a function of energy. While only one wavevector at each energy was expected due to the intra-band scattering of surface states, surprisingly, two circles corresponding to two distinct quantized wavevectors of the LDOS modulation have been identified on all three surfaces. Interestingly, these two circles merge into a single one at bias energies close to E F . The same trend is observed by performing the experiments in close proximity to a step edge ( Supplementary Fig. 1 ). The measurements reported in Fig. 1 have been acquired in the so-called constant-current mode, where the feedback loop which constantly adjusts the tip position amplifies these oscillations making them easier to be detected. However, note that the same (although less intense) behaviour is observed for measurements performed in the constant height mode ( Supplementary Fig. 2 ). The use of very different experimental conditions allows us to safely exclude the effect of artifacts introduced by the set-point parameters. The distribution of the impurities across the surface can also be ruled out as a possible origin of our findings, since the same trend emerges for measurements performed around a single impurity ( Supplementary Fig. 3 ). Moreover, experiments performed by deliberately introducing different adatoms onto the surface also provided the same results, which can thus not be link to any particular scattering centre. As a final remark, we would like to point out that a spatially resolved analysis shows the additional ring intensity being mainly located around impurities, where strong oscillations are visible and many out-of-equilibrium effects can thus take place ( Supplementary Fig. 4 ). Figure 1: Spectroscopic mapping of charge waves. ( a – i ) d I /d U maps with respective FT images obtained at different energies on Cu, Ag and Au. Two distinct rings in FT images merging into a single one at energies close to E F are visible on all three surfaces. Low row shows energy-wavevector dispersion relations of two rings for ( j ) Cu, ( k ) Ag and ( l ) Au. Data have been obtained by analysing the FT QPI pattern at different energies. Red points correspond to the surface-state dispersion. Black points correspond to the additional oscillations with wavevector denoted as k EH . Below the onset of the surface states, wavevectors corresponding to bulk states can be detected for Cu and Ag. The error bars have been calculated according to the procedure described in the Methods section. Full size image To get a better insight into the origin of these two distinct modulations, FT d I /d U maps have been quantitatively analysed by measuring the radial average for each circle at different energies (line sections can be found in Fig. 2c and in Supplementary Fig. 5 ), which was further fitted by two Gaussian curves. The obtained energy dispersion relations are reported in Fig. 1j–l . Above the onset of the surface states, two distinct wavevectors appear at each energy: k SS , which corresponds to surface states, and k EH . Their strictly simultaneous appearance demonstrates that the origin of the second ring revealed by FT d I /d U maps is intimately related to the presence of the surface state. Although quantitatively different in Cu, Ag and Au, the energy dispersion relation of k EH shows features common to all the three noble metal surfaces: (i) a notable dispersion can be detected only below the Fermi level, where for each energy we have k EH > k SS ; (ii) almost no dispersion can be measured at energies above E F where the second ring always appears close to the surface state Fermi wavevector k EH ≈ k F SS ; and (iii) the k SS and k EH energy dispersion relations always intersect each other at the Fermi level. These similarities point into the direction of a general physical process underlying our observations that is not related to the peculiar electronic structure of one of the systems. Similar observations assigned the second ring to bulk states [29] , [30] , a statement in contradiction with both photoemission data and ab initio calculations [17] , [27] . 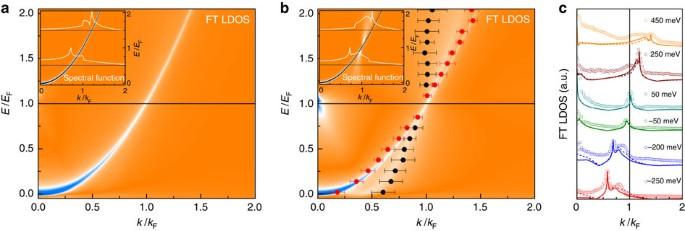Figure 2: Leading term provided by injected quasiparticles. (a,b) FT LDOS and underlying many-body spectral function (inset) for the conventional 2DEG and the 2DEG formed by surface-state electrons, respectively. The latter case is accompanied by the experimental data acquired for the Cu(111) surface and shown inFig. 1j. For comparison with the experimental data, we plot the FT LDOS as a function ofk=p/2, wherepis the magnitude of the reciprocal-space vector used in the formulas. In the insets, solid white lines show the spectral function as a function of the wavevectorkatE=0.5EFand 1.5EFin logarithmic scale. (c) FT LDOS as a function ofk=p/2 at a fixed energyEwith (dashed lines) and without (solid lines) the background contribution of ref.24in comparison with radially averaged line sections (open circles) as measured at different bias voltages for the Cu(111) surface. All the data are presented in relative units in order to underline the common nature of the considered phenomenon. Figure 2: Leading term provided by injected quasiparticles. ( a , b ) FT LDOS and underlying many-body spectral function (inset) for the conventional 2DEG and the 2DEG formed by surface-state electrons, respectively. The latter case is accompanied by the experimental data acquired for the Cu(111) surface and shown in Fig. 1j . For comparison with the experimental data, we plot the FT LDOS as a function of k = p /2, where p is the magnitude of the reciprocal-space vector used in the formulas. In the insets, solid white lines show the spectral function as a function of the wavevector k at E =0.5 E F and 1.5 E F in logarithmic scale. ( c ) FT LDOS as a function of k = p /2 at a fixed energy E with (dashed lines) and without (solid lines) the background contribution of ref. 24 in comparison with radially averaged line sections (open circles) as measured at different bias voltages for the Cu(111) surface. All the data are presented in relative units in order to underline the common nature of the considered phenomenon. Full size image Theoretical description To describe the scattering-induced LDOS oscillations, which are considered as a leading contribution to the QPI maps, we start from the Dyson equation of quantum scattering theory, corresponding to the elastic scattering of a quasiparticle with the energy E off a point defect with the scattering potential V ( r ). Further, following the ideas of refs 20 , 21 , 22 , we consider the free-motion Green function G ( r , r ′; E ) describing the quasiparticle propagation in the absence of the potential V ( r ) as the interacting Green function of many-body perturbation theory defined as where the non-interacting Green function G 0 ( r , r ′; E ) is built on the Hartree states, , of the considered 2DEG formed by surface-state electrons. Here E SS and are the surface-state band width and effective mass, respectively (atomic units e 2 = ħ = m e =1 are used). The complex and energy-dependent self-energy entering equation (2) incorporates all many-body exchange and correlation effects and allows one to bring into the QPI description the lifetime and renormalized dispersion of scattering electrons and holes. Since the 2DEG under study is homogeneous and isotropic, in k -space the interacting Green function can be cast into the form given by . The many-body spectral function, , which is essentially the imaginary part of G , presents the density of excited states contributing to the quasiparticle propagation. The quasiparticle peak of A ( k , E ) is of Lorentzian form with the peak position and width corresponding to the quasiparticle energy and inverse lifetime, respectively. However, the self-energy effects are generally not reduced to the quasiparticle picture, since besides the quasiparticle peak the many-body spectral function can acquire other features with lower intensities. Thus, we calculate A ( k , E ) in such a way that allows us to retain, as far as possible, all the features of the spectral function for FT LDOS calculations, rather than focusing on the Lorentz peak only. We model the self-energy by a G 0 W 0 formula with the screened Coulomb interaction that properly takes into account the peculiarity of the 2DEG residing on the noble metal (111) surfaces. In contrast to a conventional 2DEG, where in the long-wave limit (the transfer momentum q →0) the plasmon dispersion is described by (see ref. 31 ), in the considered 2D electron system the collective-excitation mode has a linear dispersion due to screening by the underlying three-dimensional electron system [25] . This mode is the aforementioned ASP, which was predicted to exist at metal surfaces with a partly occupied surface-state band [25] , [26] and was recently observed on Be [32] , Cu [33] , [34] and Au [35] , [36] surfaces by electron-energy-loss spectroscopy. Finally, to solve equation (1) without loss of generality, we considered a point-like potential V ( r )= V 0 δ ( r ). As a result, the scattering-induced part δG s can be rewritten as , where the k -independent T -matrix is defined as . For direct comparison with the experimental data, we calculate the FT LDOS defined as with i being the unit vector directed along the x axis, that is, the scalar product ( k , i )= k x . Further calculation details are given in Supplementary Note 1 . As a reference point, we start from the conventional 2DEG ( Fig. 2a ). In this case, the spectral function has a hardly visible satellite peak as compared with the quasiparticle one. As a consequence, only the surface-state band is well defined in the FT LDOS. The finite quasiparticle lifetime leads to a smoothing of the FT LDOS singularities and a faster reduction of the amplitude of LDOS oscillations in real space. Similar results can be obtained with a Lorentz-type spectral function containing the quasiparticle peak only. The case of surface-state electrons at noble metal (111) surfaces differs drastically. As seen in the insert in Fig. 2b , a clear satellite peak is observed in the spectral function, producing an additional band in the FT LDOS shown in Fig. 2b . This band intersects the surface-state band at the Fermi energy and has the dispersion, which can be reduced to the form of at a given energy E , where k Sat corresponds to the satellite dispersion gained from the spectral function calculations. In general, the behaviour of k EH ( E ) as compared with k SS ( E ) is in accord with the experimental observations described above. As seen in Fig. 2b , below the Fermi energy the theoretical k EH ( E ) curve agrees well with the experimental data ( Fig. 2c ). Nevertheless, above the Fermi level the calculated k EH ( E ) dispersion notably deviates from the experimentally determined one. In our attempt to overcome this discrepancy, we investigated a possible role played by the background contribution. We started from the latter evaluated according to ref. 24 as the tunnelling current with a coefficient depending on tip–sample distance and work function. In our calculations of the tunnelling current required by the formula , where U is the bias voltage and B ( E , U ) is the barrier factor ( Supplementary Note 2 ), we used the FT LDOS δN ( p , E ) shown in Fig. 2b . We found that below E F the background term increases the intensity of the satellite-derived peak and slightly shifts its position away from the k SS ( E ) peak. Above the Fermi energy, the tunnelling current changes its sign, and the background term generates a gap near k F . However, it neither redistributes a spectral weight from the calculated k EH ( E ) curve to the experimentally determined position nor leads to the appearance of a feature around the Fermi wavevector comparable with the experimental one. Alternatively, the background term can be described as follows. The imaging process can be considered as that initiated by injecting an electron or a hole into the surface-state band in an initial state i with the energy E i and wavevector k i defined by the applied bias voltage. In providing the appearance of the leading term, this injected electron (hole) decays into an energetically lower state f with the wavevector k f and the energy E f within the energy range between E i (− E i ) and E F , thereby transferring the momentum q = k i − k f to the system. It results in the creation of an electron–hole pair. The excitations of these quasiparticles occur in an incoherent way, thus not allowing any possible interference arising from the superposition of initial and final states. However, once generated, each secondary quasiparticle, such as the primary one, may move across the surface and experience elastic reflection from impurities, thereby establishing corresponding standing waves. To model the experimental data within the injection-decay scenario described above, we consider that the distribution of secondary quasiparticles produced in a non-equilibrium steady decay process within the energy interval between −| E i | and | E i | is governed by the Fermi’s golden rule ( Supplementary Note 3 ), where the probability of decay from an electron state i into the state f is expressed as: where W is the screened dynamical Coulomb interaction ( Supplementary Note 4 ), f k is a Fermi factor, f P i→f ( k f )=1, and Γ i −1 is the quasiparticle lifetime. The upper panel of Fig. 3 shows the calculated distribution P i→f ( k f ) for the Cu(111) surface state (taken as an example) as a function of k f for initial energies equal to (a) the onset of the surface state ( E i =−440 meV), (b) E i =−230 meV and (c) E i =+500 meV. While (a) and (b) correspond to hole injection, (c) refers to electron injection, thereby spanning the entire excitation scenario. As can be seen in Fig. 3a , for a hole with k i =0 the probability distribution is independent of the final wavevector azimuthal angle and grows gradually with increasing k f reaching its maximum value in the proximity of the Fermi circle. When increasing k i , a significant azimuthal dependence of P i→f ( k f ) sets in, as can be recognized in Fig. 3b . Nevertheless, P i→f ( k f ) maintains its maximum at the Fermi circle at any azimuthal angle. The picture becomes strikingly different at positive injection energy ( Fig. 3c ), where one clearly sees how P i→f ( k f ) is extremely inhomogeneous and sharply peaked along the dotted line determined by the ASP dispersion. 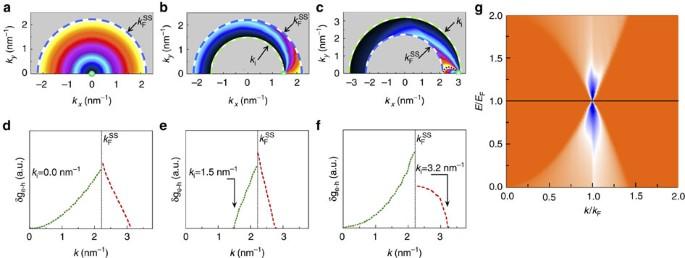Figure 3: Background contribution of secondary quasiparticles. (a–c) Calculated probability distributionPi→f(kf) of final states versus final wavevectorkf≡ (kx,ky) (axiskxis directed alongkiand the data for negativeky′s are symmetrical) of inelastic decay for a quasiparticle initially injected into the Cu(111) surface-state band at energyEiof −440, −230 and +500 meV, respectively. In each panel, the position of the initial-state wavevector is shown by green dot. Blue- and green-dashed lines highlight the Fermik=kFSSandk=kisemicircles, respectively, delimiting available regions of the final states to decay in the momentum space. (d–f) Corresponding background contribution of secondary electrons (red-dashed line) and holes (green dot line) forming the excited (e–h) pairs, generated during the inelastic decay of a quasiparticle initially injected in the state withki. (g) Background contributionof secondary quasiparticles to the FT QPI pattern versusk=p/2 and initial-quasiparticle energy. Figure 3: Background contribution of secondary quasiparticles. ( a – c ) Calculated probability distribution P i→f ( k f ) of final states versus final wavevector k f ≡ ( k x , k y ) (axis k x is directed along k i and the data for negative k y ′s are symmetrical) of inelastic decay for a quasiparticle initially injected into the Cu(111) surface-state band at energy E i of −440, −230 and +500 meV, respectively. In each panel, the position of the initial-state wavevector is shown by green dot. Blue- and green-dashed lines highlight the Fermi k = k F SS and k = k i semicircles, respectively, delimiting available regions of the final states to decay in the momentum space. ( d – f ) Corresponding background contribution of secondary electrons (red-dashed line) and holes (green dot line) forming the excited ( e – h ) pairs, generated during the inelastic decay of a quasiparticle initially injected in the state with k i . ( g ) Background contribution of secondary quasiparticles to the FT QPI pattern versus k = p /2 and initial-quasiparticle energy. Full size image To take into account all possible electron–hole pairs and their contributions to the background term, in the spirit of the formula for the tunnelling current mentioned above, we performed integration of the self-interfering patterns δN produced by these secondary quasiparticles (for simplicity, each of them has been represented by a δ -function in reciprocal space) over the available phase space with P i→f ( k f ) as the weighting factor: where the difference between electron ( k e ) and hole ( k h ) wavevectors is restricted as k h − k e = k i − k f ( Supplementary Note 3 ). The evaluated term is reported in Fig. 3d–f at selected k i ′s. A clear peak in the vicinity of k F SS is observed in these curves, apart from a strong enhancement on the right side for electrons (red-dashed line in Fig. 3f ) caused by the ASP excitation. This peak becomes broader as U moves away from the zero bias voltage, as is distinctly seen in Fig. 3g . Thus, the resulting background term can already ensure a noticeable peak comparable with the experimental observations. Apparently, this very term provides the primary contribution to the FT QPI feature appearing at the Fermi wavevector for energies above E F . Overall, our results show that the decay mechanisms of excited electrons and holes can give rise to charge density oscillations. More generally, our approach demonstrates that STM measurements can be used to provide direct access into many-body interactions at the atomic scale, further expanding the capabilities of this experimental technique. Many-body effects and their influence on quantum coherence are known to be relevant in several exciting area of condensed matter physics, such as superconductivity and quantum information, where they give rise to remarkable macroscopic properties. However, these effects are usually challenging to be measured, especially with spatial resolution. Consequently, using a local probe to visualize them is expected to give important contributions to understanding unconventional physical properties on a microscopic scale. Experimental details The experiments have been performed in an ultrahigh vacuum system equipped with a cryogenic STM operated at T =4.8 K. Single crystals have been prepared with several cycles of Ar + sputtering and subsequent annealing at T =700 K. To exclude artifacts, d I /d U maps have been acquired by lock-in technique in both constant-current ( Fig. 2 in the main text) and constant height mode ( Supplementary Fig. 1 ). The bias voltage modulation was in between 1 and 20 meV (r.m.s.) at a frequency of 793 Hz, with the amplitude progressively increasing with the scanning bias. Before Fourier transformation, the average value has been subtracted to each d I /d U map. At each energy, the k -vector has been obtained considering a Gaussian curve fitting each peak in the radially averaged line section of FT d I/ d U maps. The error bars appearing in Figs 1 and 2 correspond to the full width at half maximum of the Gaussian curves. How to cite this article: Sessi, P. et al . Direct observation of many-body charge density oscillations in a two-dimensional electron gas. Nat. Commun. 6:8691 doi: 10.1038/ncomms9691 (2015).